Draft genome sequence of the Tibetan antelope The Tibetan antelope ( Pantholops hodgsonii ) is endemic to the extremely inhospitable high-altitude environment of the Qinghai-Tibetan Plateau, a region that has a low partial pressure of oxygen and high ultraviolet radiation. Here we generate a draft genome of this artiodactyl and use it to detect the potential genetic bases of highland adaptation. Compared with other plain-dwelling mammals, the genome of the Tibetan antelope shows signals of adaptive evolution and gene-family expansion in genes associated with energy metabolism and oxygen transmission. Both the highland American pika, and the Tibetan antelope have signals of positive selection for genes involved in DNA repair and the production of ATPase. Genes associated with hypoxia seem to have experienced convergent evolution. Thus, our study suggests that common genetic mechanisms might have been utilized to enable high-altitude adaptation. The Tibetan antelope (TA; Pantholops hodgsonii ) is a large, endemic artiodactyl that lives at elevations of 4,000–5,000 m on the Tibetan Plateau [1] . This habitat has a low partial pressure of oxygen (PO 2 ) and a high level of ultraviolet radiation. Non-native animals such as humans that visit such high-altitude regions may experience life-threatening acute mountain sickness. In contrast, the TA, which has survived for millions of generations on the plateau, can run at up to 80 km per hour for several hours in this low oxygen condition. These observations indicate that the TA must have evolved exceptional mechanisms to adapt to this extremely inhospitable habitat [2] , yet the genetic bases of such adaptations remain unknown. Sequencing the TA genome will undoubtedly facilitate the discovery of potential molecular mechanisms of high-altitude adaptation. Herein, using the next-generation, massively parallel sequencing technology—Illumina Genome Analyser—we report our generation and assembly of a draft genome for the TA. Further, we compare the TA genome to that of the American pika ( Ochotona princeps ), which is also native to high altitudes [3] , to study the potential genetic basis for high-altitude living. Shotgun sequencing and de novo assembly Genomic DNA extracted from a male TA at Kekexili National Nature Reserve, Qinghai-Tibetan Plateau was subjected to shotgun sequencing using the Illumina short paired-end sequencing platform. We prepared 19 pair-end libraries spanning several insert sizes (from 165 to 20 Kb, Supplementary Table S1 ) to generate short pair-end reads. A total of 187 Gb of sequence data was generated for paired-end read lengths of 45 and 75 bp. Generated reads were assembled using a pipeline designed for short paired-end reads [4] . We improved the quality of assembly by adding 90 bp pair-end reads of a 165 bp insert size for contig-assembly, and 45 bp pair-end reads of the 20 Kb insert size for scaffold assembly. Our final assembly had an N50 contig size of 18.6 Kb and an N50 scaffold size of 2.76 Mb ( Supplementary Table S2 ). We evaluated genomic coverage by sequencing a set of 5,547 expressed sequence tags (ESTs) followed by BLAT [5] . About 95% of the ESTs mapped to the assembly ( Supplementary Table S3 ). While considering the remaining 5% of unmapped ESTs that had an equivalent gene distribution, we estimated that the genome-size was 2.75 Gb, which was slightly smaller than that of the cow (2.92 Gb) (ref. 6 ). We then used SOAPALIGNER [7] to realign all usable sequencing reads onto an assembly to evaluate the single-base accuracy of the assembled genome. The peak sequencing depth was 53X and >97% of the assembled sequences were covered by over 20 reads ( Supplementary Fig. S1 ). The GC content pattern of the TA was similar to that of the cow, horse, human and mouse. Only a minor fraction of the TA genome had GC content <20% (0.01%) or >80% (0.2%) ( Supplementary Fig. S2 ). Thus, the de novo genomic assembly for the TA covered high reads and it was not strongly affected by GC-biased non-random sampling. Accuracy of the scaffolds was evaluated by aligning them with the 26 available sheep BAC clones and the cow genome. Fine genomic synteny was detected ( Supplementary Fig. S3 ). The trinucleotide class of simple sequence repeats in TA was usually <12 bp ( Supplementary Fig. S4a ) and this was similar to that of the cow ( Supplementary Fig. S4b ). Whole-genome alignment of TA with the cow and human showed 635 Mb of shared sequences. Of the remainder, 499 Mb were shared between TA and cow, which was much higher than that between TA and human (107 Mb) or between cow and human (72 Mb) ( Supplementary Fig. S5 ). We identified 2.2 million heterozygous single-nucleotide polymorphisms (SNPs) along the assembled TA genome and found two peaks in the distribution of SNP density ( Fig. 1 ). 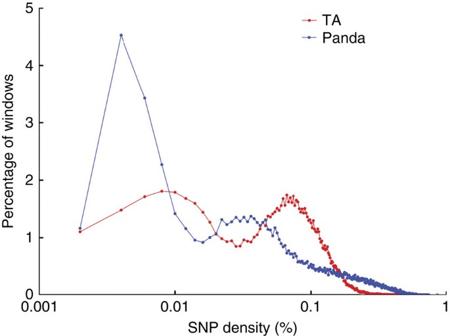Figure 1: Comparison of heterozygous SNP density between genomes of panda and Tibetan antelope. Heterozygous SNPs between two sets of chromosomes of the panda and Tibetan antelope diploid genomes were identified. Non-overlapping 50 Kb windows were chosen and the heterozygosity density was calculated. Figure 1: Comparison of heterozygous SNP density between genomes of panda and Tibetan antelope. Heterozygous SNPs between two sets of chromosomes of the panda and Tibetan antelope diploid genomes were identified. Non-overlapping 50 Kb windows were chosen and the heterozygosity density was calculated. Full size image To predict the number of genes in the TA genome, we used both evidence-based and ab inito methods. Considering the finest gene set of human and the closet phylogenic distance of cow to TA, 22,389 human protein-coding genes and 20,892 protein-coding cow genes were projected for the TA genome, and we predicted 16,995 and 18,957 gene models, respectively. This method obtained conserved gene models among mammals only. To predict species-specific genes, we used GENSCAN [8] , AUGUSTUS [9] and GLIMMERHMM [10] with model parameters trained on human and cow genomes, and predicted 53,608, 51,944 and 23,402 gene models, respectively. We integrated all five gene-sets to obtain a final gene-set of 21,426 protein-coding genes ( Supplementary Table S4 ). The length distribution of genes, length of coding sequences (CDS), exon length, intron length, CDS GC ratio and distribution of exon number per gene for TA were compared with those of cow, horse, human and mouse. No obvious difference in any of these measures was seen for the TA ( Supplementary Figs S6 and S7 ). Genome and genome evolution Compared with protein-coding genes of eight other mammals (cow, human, mouse, rat, chimpanzee, macaque, horse and dog), we detected 12,077 orthologous clusters that were shared between all the organisms. Further, 357 orthologous clusters were shared only between the TA and cow; these may have represented ruminate-specific genes ( Fig. 2 ). Gene Ontology (GO) function categories were shown in Supplementary Table S5 . Transposable elements comprised ~37% of the TA genome. The majority of known repeats present in the cow were found in the TA genome and the total number of elements in each major category was similar between the two genomes ( Supplementary Table S6 ). Among major repeat families ( Supplementary Table S7 ), the non-LTR (long terminal repeat) retrotransposons accounted for >80% of the repeats and two, major, long interspersed elements (RTE-BovB and L1) were active. 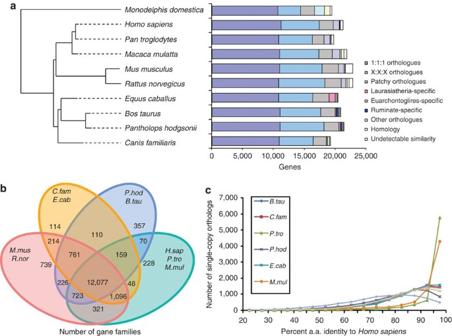Figure 2: Evolution of gene clusters among mammals. (a) Phylogeny and the distribution of gene clusters among the mammals. (b) Orthologs shared between rodents (mouse and rat, red colour), ruminates (TA and cow, blue colour), primates (human, chimpanzee and macaque, dark turquoise colour) and non-Artiodactyla laurasiatherians (horse and dog, orange colour) on the basis of a representative gene in at least one of the grouped species. (c) Protein identity between other mammals and humans for strictly conserved single-copy orthologs. Figure 2: Evolution of gene clusters among mammals. ( a ) Phylogeny and the distribution of gene clusters among the mammals. ( b ) Orthologs shared between rodents (mouse and rat, red colour), ruminates (TA and cow, blue colour), primates (human, chimpanzee and macaque, dark turquoise colour) and non-Artiodactyla laurasiatherians (horse and dog, orange colour) on the basis of a representative gene in at least one of the grouped species. ( c ) Protein identity between other mammals and humans for strictly conserved single-copy orthologs. Full size image Ancestral homologous synteny blocks (aHSBs) for the common ruminant ancestor of the cow and TA were reconstructed by identifying shared homologous synteny blocks (HSBs). The human genome was used as the outgroup to determine if the adjacent regions were present in the ruminant common ancestor. The cow and TA shared 1,597 HSBs with lengths >150 Kb, which corresponded to 1,434 TA scaffolds. These HSBs contained 95% of the assembled TA genomic sequence and covered all 29 autosomes and the X chromosome of the cow ( Supplementary Table S8 ). We then reconstructed 138 ruminant aHSBs, which represented the ancestral sequence order and orientation of the Cow-TA HSBs. Five of the aHSBs (6, 7, 47, 76 and 96) corresponded to complete cow chromosomes (BTA 2, 3, 12, 20 and 25, respectively) and the size of the longest aHSB (ruminant aHSB 6) was 138 Mb long and consisted of 75 TA scaffolds that spanned all of cow chromosome 2. Among the 1,434 TA scaffolds that aligned to the cow genome, 92 (6%) split into more than one HSB, of which 87 had HSBs that mapped to different ruminant aHSBs; five had HSBs that mapped to different positions in the same ruminant aHSB ( Supplementary Table S9 ). These 92 scaffolds may have been chimeras or sequences containing authentic TA-specific breakpoints. By mapping cow and human genome sequences to the reconstructed ruminant aHSBs, we recovered 13 cow-specific and 280 primate- or artiodactyl-specific chromosomal evolutionary breakpoint regions ( Supplementary Table S9 ; examples in Supplementary Fig. S8 ). The fragmented nature of the TA assembly suggested that additional chromosomal evolutionary breakpoints may exist. Our breakpoint data demonstrated that large insert mate-pair libraries (such as the 20 Kb library) were very powerful tools for assembling sequence scaffolds. Potential molecular mechanism of high-altitude adaptation The genome of the TA was compared with the draft genome of the American pika, another high-altitude species [3] . Positively selected genes in the TA and pika were detected by assigning branches leading to the American pika and TA as forward branches ( Supplementary Data sets 1 and 2 ). They were enriched in ATPase and DNA repair categories ( Table 1 ). The TA and pika shared 76 genes that showed signals of positive selection. GO analysis identified 12 genes involved in the regulation of angiogenesis ( P =0.018), folic acid and derivative biosynthetic processes ( P =0.036), as well as DNA repair ( P =0.046). Table 1 GO enrichment analysis of positive selection genes in the branch leading to Tibetan antelope and pika, respectively. Full size table Among the 247 hypoxia genes examined, seven showed significant signals of convergent/parallel evolution ( P <0.05): ADORA2A , CCL2 , ENG , PIK3C2A , PKLR , ATP12A and NOS3 . As the American pika genome was a draft production, we also resequenced these seven genes in the Tibetan pika ( Ochotona curzoniae ), which occurs on the highest plateau in the world [11] ; we detected convergent/parallel evolved amino acid sites in both species of pika and the TA. Segmental duplication (SDs) is a common means of increasing gene copy number. We identified 4,640 duplicated fragments that represented recent SDs (>90% identity, >1 Kb length) in the TA genome via self-alignment. These comprised 22.6 Mb of sequences, which was less than that seen in the cow ( Supplementary Table S10 ). The TA and cow shared the majority of the SDs. TA-specific SDs were related to energy metabolism such as NAD- and NADH-binding (GO:0051287) and ATP synthesis (GO:0006754 and GO:0015986) ( Supplementary Table S11 ). Gain and loss of genes in gene families could have had a role in adaptive evolution. The size of each gene family was determined by comparing the TA gene set with those of nine other mammals (cow, dog, horse, human, chimpanzee, macaque, opossum, mouse and rat) obtained from Ensembl. These analyses facilitated inferences into the expansion or contraction of each family ( Supplementary Fig. S9 ). For TA, a large fraction of lost genes involved olfactory receptors and immunity. In contrast, genes that had functions associated with mitochondrial membranes, and, thus, potentially metabolic functions, had gains ( Supplementary Table S12 ). Many expansions of gene families were related to energy metabolism (listed in Table 2 ). Table 2 Outstanding GO enrichment of expanded gene families for the Tibetan antelope. Full size table Our final assembly of the TA genome based on next-generation sequencing technology has an N50 contig size of 18.6 Kb and an N50 scaffold size of 2.76 Mb ( Supplementary Table S2 ). About 95% of the ESTs map to the assembly ( Supplementary Table S3 ). This suggests that our assembly is good enough for the following comparative genome analyses. The length distribution of genes, length of coding sequences (CDS), exon length, intron length, CDS GC ratio and distribution of exon number per gene for the TA do not obviously differ from those of the cow, horse, human and mouse ( Supplementary Figs S6 and S7 ). Correspondence in these measures indicates a high quality of annotation for gene structure in the genome of the TA. The pattern of heterozygous SNPs along the assembled TA genome is similar to that of the panda [4] ( Fig. 1 ). The same as panda, this pattern may indicate a bottleneck in the TA population caused by human hunting during the past tens of years. Compared with eight other mammals (cow, human, mouse, rat, chimpanzee, macaque, horse and dog), 12,077 orthologous clusters are shared between all the organisms, and 357 are shared only between the TA and cow. The latter cluster may represent ruminate-specific genes ( Fig. 2 ). Positively selected genes in TA are in the ATPase and DNA repair categories ( Table 1 ). These categories appear to be biologically relevant to living at high altitudes. ATPase genes have a role in providing energy. DNA repair genes may need to be more efficient given exposure to high levels of ultraviolet radiation. In addition, segmental duplications ( Supplementary Table S13 ) and expansions of gene families ( Table 2 ) also relate to energy metabolism. Thus, positive selection and expansion of gene families involved in energy metabolism appear to have an important role for TA via efficiently providing energy in conditions of low PO 2 . Positively selected genes shared by the TA and pika involve the regulation of angiogenesis ( P =0.018), folic acid and derivative biosynthetic processes ( P =0.036), as well as DNA repair ( P =0.046). Folic acid, required for the synthesis and repair of DNA and the production of healthy red blood cells, aids in preventing anaemia [12] . Therefore, gene term GO:0009396 (folic acid and derivative biosynthetic process) may reflect gene selection for both low PO 2 and high ultraviolet radiation. Seven of 247 hypoxia genes have signals of parallel/convergent sequence evolution in TA and pika. Several of these are particularly interesting because of their functional implications. For example, PKLR encodes pyruvate kinase, which catalyses the transphosphorylation of phosphoenolpyruvate into pyruvate and ATP, a rate-limiting step in glycolysis. Parallel/convergent evolution of this gene may reflect the importance of glycolysis in energy metabolism for survival in hypoxic, high-altitude environments. Another gene, NOS3 (endothelial nitric oxide synthase), is a critical mediator of cardiovascular homoeostasis. It regulates the diameter of blood vessels and in doing so maintains an antiproliferative and antiapoptotic vascular environment [13] . Parallel/convergent evolution of this gene suggests that high-altitude adaptation involves the use of nitric oxide to regulate the diameter of blood vessels, which increases blood flow, thus allowing tissues to attain more oxygen. In extremely high environments, low PO 2 can result in a precipitous reduction in O 2 saturation in arterial blood. At 4,000 m altitude, PO 2 of inspired air is ~60% of that at sea-level. Thus, in the absence of adaptations or compensatory physiological mechanisms, O 2 transport to tissues is severely compromised and this influences metabolism and the capacity to sustain physical activity [14] , [15] . Analyses of gene sequence convergence indicate that indigenous montane animals may use two major strategies to deal with hypoxia: (1) placing increased reliance on glycolysis; and (2) regulating blood vessel diameter, specifically through nitric oxide. High ultraviolet and especially hypoxia are the most important ecological factors restricting the viability of high-plateau animals. Native animals on the plateau that have survived there over thousands of years must have developed adaptive mechanisms to address harsh environmental stresses during their long history [16] . Previous studies on Tibetan people identified some of the genetic bases for adaptation to a high-altitude environment [17] , [18] , [19] . Considering that Tibetans arrived on the plateau only 2,750 years ago [17] , this relatively short time scale suggests that their adaptation to the highland may be ongoing and not fully integrated genetically. Domestic yaks yield some clues for highland adaptation [20] . However, artificial selection may confuse such results. Unlike Tibetans and domestic yak, native highland animals, such as the TA and pika, have adapted to this harsh environment for millions years. Thus, the study of genomes of native highland animals should provide a more complete blueprint to the genetic mechanisms of highland adaptation. Our study obtains a draft genome for the TA and identifies common themes of positive selection involved in DNA repair, ATPase function, angiogenesis and hypoxia, and parallel/convergent sequence evolution in genes that respond to hypoxia in TA and pikas. These discoveries potentially identify common genetic mechanisms of adapting species to harsh highland environments. Unfortunately, no genome is available from a sister species of the TA that is native to low altitudes. This absence of data precludes a genome-wide comparison. Thus, we cannot exclude the possibility that some genetic differences between the TA and cow may be due simply to divergence as a function of time and not high-altitude adaptation. Additional genomes will allow testing for adaptation. Genome sequencing and de novo assembly We constructed 19 paired-end DNA libraries with insert sizes of about 150 bp, 500 bp, 2 kb, 5 kb, 10 kb and 20 kb. For libraries of insert size longer than 1 kb, the desired DNA fragments were circularised by self-ligation. After being randomly fragmented, fragments that crossed the ligation boundaries were then enriched using magnetic beads with biotin and streptavidin. Paired-end sequencing was done on the Illumina Genome Analyser platform following the manufacturer’s instructions. Fluorescent images were processed into sequences using the Illumina data processing pipeline. The genomic sequence was assembled from the short reads using SOAPDENOVO [21] . Contigs were constructed by adopting the de Bruijn graph data structure [22] from short reads (mainly short insert size-reads) without using paired-end information. Reads were then realigned to the contig sequences, and paired-end relationships between the reads allowed linkage between the contigs. Scaffolds were constructed by iteratively adding different class insert size of paired-ends sequentially from short to long. To fill intra-scaffold gaps, we used paired-end information to retrieve read pairs that had one read well aligned on the contigs and the other read located in a gap region. We then performed a local assembly with the collected reads. Genome annotation The TA protein-coding genes were annotated by combining evidence-based gene prediction and de novo gene prediction. For evidence-based gene prediction, the cow and human genes (Ensembl release 56) were projected onto the TA genome, and gene loci were defined using both sequence similarity and information on whole-genome synteny. De novo gene prediction was performed using GENSCAN [8] , AUGUSTUS [9] and GLIMMERHMM [10] . Finally, a consensus TA gene-set was created by merging the gene-sets from all of these predictions. Known transposable elements were identified using REPEATMASKER (v.3.2.6) and the REPBASE transposable element library (v.2008-08-01) [23] . Highly divergent transposable elements were identified with REPEATPROTEINMASK after aligning the genome sequence to curated transposable element-related proteins. A de novo repeat library was constructed using REPEATMODELLER. Details of sequencing, assembly and annotation are given in Supplementary Methods . Construction of HSBs between cow and TA The cow genome assembly (UMD 3.0) was aligned with the de novo TA assembly (2,598 TA scaffolds with length >10 Kb) using LASTZ ( http://www.bx.psu.edu/miller_lab/dist/README.lastz-1.02.00/README.lastz-1.02.00a.html ). Alignment nets, which were putative orthologous regions, were then created using tools available at the UCSC Genome Browser [24] . HSBs were constructed by merging colinear alignments [25] . We discarded HSBs of length ≤150 Kb. Reconstruction of ancestral HSBs aHSBs of the ruminant common ancestor of cow and TA were reconstructed by predicting the ancestral order and orientation of HSBs using their observed adjacencies in extant species. To help resolve the ambiguity of the ancestral configuration, we used matches of the HSBs to the human genome (NCBI36/hg18 assembly) as outgroup information. We connected adjacent cow-TA HSBs into aHSBs when each ancestral adjacency was supported by either the organization within the cow and human genomes, or the TA and human genomes. Ancestral HSBs were separated when adjacencies of the cow-TA HSBs were not supported by human genome organization. Comparison of sheep BAC to cow and TA genome Twenty-six BAC clones from sheep chromosome 20 with complete sequences were identified in the NCBI database (accession number: FJ985852.1- FJ985877.1). Following alignment to the TA genome, 16 mapped onto one TA scaffold and showed fine genomic synteny. We then mapped the TA scaffold sequence to the cow genome and obtained an alignment. The other BAC sequences, except for two sequences, mapped to other scaffolds. Whole-genome alignment Pairwise whole-genome alignment among TA, cow and human was carried out using LASTZ ( http://www.bx.psu.edu/miller_lab/dist/README.lastz-1.02.00/README.lastz-1.02.00a.html ), with the parameters: C =2, T =2, H =2,000, Y =3400, L =6000, K =2200. CHAIN/NET was used for post-treatment. The TA genome was masked with REPEATMASKER ( www.repeatmasker.org ) with the REPBASE and de novo constructed libraries using PILE and REPEATMODELER and TRF tandem repeats of period ≤12. The cow (BTA4.0) and human (hg18) repeat-masked genomes were download from UCSC ( http://genome.ucsc.edu ). A three-way, whole-genome multiple alignment including human (hg18), cow (BTA4.0) and TA was conducted by MULTIZ ( http://multiz.com ), guided by the topology of their species tree. The human genome was set as the reference and for input pairwise alignments the human versus cow and human versus TA alignments were generated. Whole-genome assembly comparison methods were used to identify SDs [26] . Self-alignment of each genome was implemented by LASTZ with parameters T =2, Y =9,400. We defined a SD as two sequences longer than 1 kb with an identity >90%, but <98% to exclude potential improperly assembled allelic variants that may possibly reside in the ‘draft’ genome. Adaptive evolutionary analyses We used the TREEFAM methodology [27] to define a gene family as being a group of genes descendent from a single gene in the last common ancestor. We applied a pipeline to cluster individual genes into gene families and performed phylogenetic analysis as below. (1) Data preparation: protein-coding genes from 10 mammalian species were used in this analysis; we retained the longest transcript isoform only for each gene and only considered proteins larger than 50 amino acids. (2) Pairwise relationship assignment (graph building): we performed BLASTP on all protein sequences against the database containing protein data of all of the species with an E -value cutoff of 10 −5 and conjoined fragmented alignments for each gene pair using SOLAR ( http://treesoft.svn.sourceforge.net/viewrc/treesoft/branches/dev/solar ); we assigned a connection (edge) between two nodes (genes) if more than 1/3 of the region was aligned in both genes; an H-score ranging from 0 to 100 was used to weigh the similarity (edge); for two genes, G1 and G2, the H-score was defined as score (G1G2)/ max(score(G1G1), score(G2G2)), (score=BLAST raw score). (3) Gene-family construction: we used the average distance for the hierarchical clustering algorithm, requiring the minimum edge weight (H-score) to be >5 and the minimum edge density (total number of edges/theoretical number of edges) to be larger than 1/3; clustering for a gene family was terminated when the presence of one or more outgroup genes was detected. (4) Phylogeny and orthology analyses: we performed multiple alignments of protein sequences for each gene family using MUSCLE [28] and converted the protein alignments to CDS alignments using a Perl script; we built phylogenies using TREEBEST ( http://treesoft.sourceforge.net/treebest.shtml ), which took advantage of both codon-based and aa-based algorithms (nj-dn, nj-ds, nj-mm, phyml-aa and phyml-nt) and adjusted them to the topology of the species tree to form a more accurate consensus tree. We inferred orthologous and paralogous gene relationships from the gene tree. We inferred the rate and direction of change in gene-family size for the TA, cow, dog, human, mouse and rat. The average rate of gene turnover across the animals, which was the rate at which the size of the gene family was expected to expand or contract over time due to the gains or losses, was estimated first. Using the phylogeny, and while taking into account the topology and branch-lengths taken, we inferred changes in gene-family size and its significance. We used the Ensembl ortholog_one2one gene database [29] for each pair of species including the cow, dolphin, dog, pika, rabbit and mouse. Only those genes that were one-to-one orthologs for every pair of genomes for the six species were used. For those genes that have more than one transcript, we used the longest transcript of cow to blast the TA genome and obtain its best-hit sequence and E o value. This best-hit sequence from the TA was then used to blast the cow and TA genomes. This obtained the best-hit cow sequence and E 1 value and the second best-hit TA sequence and E 2 value. The best-hit cow sequence was expected to be the same as the cow sequence that was used to blast TA in the first step. If the values of E o and E 1 were both less than the value E 2 , we considered this gene to be an ortholog one2one for cow-TA. After these ortholog-finding treatments, KALIGN [30] was used to align the sequences. To reduce errors due to sequencing, incorrect alignments and non-orthologus regions in the alignments, we employed a previously used strategy [31] as follows: a 15-bp sliding window was used on each alignment and moved by one codon for each step to the end of the alignment. For each window, we calculated the lowest similarity of an alignment pair of the eight species within the sliding window. Aligned regions with lowest similarity (<7/15) were discarded as these may have included errors in sequence or assembly. After the deletion step, if the remaining alignment was shorter than 100 bp, then the entire alignment was discarded. After these strict treatments, our final data set contained 5,082 one-to-one orthologous genes. Alignments and consensus trees were used for posterior molecular evolutionary analysis. We used a gene-level approach based on the ratio ω of non-synonymous ( Ka or dN ) to synonymous ( Ks or dS ) substitutions rate ( ω = Ka/Ks or dN/dS ) to identify potential positive selection, using the CODEML algorithm in the PAML 4 package [32] . Branches of the TA and pika were set as forward branches. We then used the branch site model to detect positive selection. For analyses of convergent evolution, the most likely ancestral states of all internal nodes of the species tree were reconstructed by PAML. We then recorded parallel and convergent double amino acid replacements for pairwise comparison of branches leading independently to the pika and TA. The statistical significance of these amino acid changes was tested with the method developed by Zhang and Kumar [33] . Human NCBI EntrezGene IDs were used in all analyses of gene ontology. Non-human orthologs of the human genes were retrieved from Ensembl Biomart. For uniformity of functional annotation enrichment results, we used the human NCBI EntrezGene IDs to refer to both the human genes and to their putative non-human orthologs. We used DAVID [34] , [35] as a functional annotation clustering tool for each combination of species and d N/ d S bin to group genes with shared annotations. The algorithm assigned a significance P -value, corrected for multiple testing, to each subgroup representing a gene ontology annotation within the cluster and an enrichment score to the entire cluster. The clusters with higher enrichment scores consisted of subgroups with higher significance values, and, thus, these clusters provided an integrated view of the more significantly enriched or over-represented gene functional categories within each d N/ d S bin. The enrichment score for each annotation cluster was based on the geometric mean of the P -values of the cluster’s assorted annotations. Accession codes: This Whole-Genome Shotgun project has been deposited in GenBank Genome database under the accession number AGTT00000000 . The version described in this paper is the first version, AGTT01000000 . How to cite this article: Ge, R. -L. et al . Draft genome sequence of the Tibetan antelope. Nat. Commun. 4:1858 doi: 10.1038/ncomms2860 (2013).